Sugar-mediated regulation of a c-di-GMP phosphodiesterase inVibrio cholerae Biofilm formation protects bacteria from stresses including antibiotics and host immune responses. Carbon sources can modulate biofilm formation and host colonization in Vibrio cholerae , but the underlying mechanisms remain unclear. Here, we show that EIIA Glc , a component of the phosphoenolpyruvate (PEP):carbohydrate phosphotransferase system (PTS), regulates the intracellular concentration of the cyclic dinucleotide c-di-GMP, and thus biofilm formation. The availability of preferred sugars such as glucose affects EIIA Glc phosphorylation state, which in turn modulates the interaction of EIIA Glc with a c-di-GMP phosphodiesterase (hereafter referred to as PdeS). In a Drosophila model of V. cholerae infection, sugars in the host diet regulate gut colonization in a manner dependent on the PdeS-EIIA Glc interaction. Our results shed light into the mechanisms by which some nutrients regulate biofilm formation and host colonization. Most bacterial species can form biofilms, which are multicellular communities embedded in a self-produced polymeric matrix. The ability of pathogenic bacteria to form biofilms facilitates their colonization and persistence in the host due to the evasion of the immune response and increased resistance to many antimicrobials [1] , [2] . In addition, it has been reported that dispersed cells exhibit acute virulence and efficient transmission to other hosts, indicating that an appropriate transition to planktonic cells from these sessile lifestyles is a crucial factor in their pathogenicity [3] , [4] , [5] , [6] . Thus, it is conceivable that sophisticated mechanisms should have evolved for pathogenic bacteria to regulate the transition between these two lifestyles in response to various environmental cues [7] . It has been shown that glucose and some other sugars in the environment induce the multilayer biofilm formation and the sugars promoting biofilm formation are substrates of the phosphoenolpyruvate (PEP):carbohydrate phosphotransferase system (PTS) in V. cholerae [7] . This multi-component system mediates the transport of various sugars including glucose in V. cholerae , and these PTS sugars are concomitantly phosphorylated during transport [8] , [9] . The PTS consists of two general components, enzyme I (EI) and histidine phosphocarrier protein (HPr) that participate in the transport of most PTS sugars, and several sugar-specific components collectively known as enzyme IIs (EIIs). EI and HPr transfer a phosphoryl group from PEP to EII components, which finally phosphorylate PTS carbohydrates during their translocation across the membrane. In addition to its role in carbohydrate transport and phosphorylation, the PTS acts as an efficient signal transduction system, which can sense the availability of carbohydrates in the environment and thereby regulates various cellular functions [10] . Phosphorylation of the PTS components usually increases in the absence and decreases in the presence of a PTS carbohydrate such as glucose [11] , [12] . Depending on their phosphorylation state, the PTS components regulate various sugar-related phenotypes by interacting with their cognate partners [13] . Although the effects of the PTS on biofilm formation have been reported in several studies [9] , [14] , [15] , the regulation mechanism of biofilm formation by the PTS has not been fully elucidated. In enteric bacteria such as Escherichia coli , EIIA Glc (encoded by crr ) is known to play multiple regulatory roles: dephosphorylated EIIA Glc inhibits non-PTS sugar permeases, such as lactose permease and stimulates the fermentation/respiration switch protein FrsA [13] , [16] , whereas only phosphorylated EIIA Glc stimulates adenylate cyclase and thus increases the concentration of cAMP [17] , which is known to suppress biofilm formation in V. cholerae [18] , [19] , [20] . An interesting difference between the E. coli and V. cholerae PTS lies in the substrate specificity of EIIA Glc . While EIIA Glc is specific for glucose in E. coli , its V. cholerae ortholog is shared among several PTS sugars, such as N -acetylglucosamine, trehalose, and sucrose as well as glucose [21] . Therefore, it could be assumed that EIIA Glc may have distinct regulatory roles in response to several PTS sugars depending on the species. Unlike in E. coli , dephosphorylated EIIA Glc of Vibrio vulnificus inhibits flagella assembly and hence motility, allowing it to efficiently consume a preferable sugar in the environment [22] , [23] . This regulation of the transition from a motile to non-motile lifestyle mediated by EIIA Glc might also act on biofilm formation processes on the abiotic or biotic surfaces. The regulatory functions of EIIA Glc on biofilm formation were suggested in V. cholerae in previous studies. EIIA Glc was shown to interact with MshH, a homolog of E. coli CsrD [14] , and a following study showed that dephosphorylated EIIA Glc activates CsrB/C turnover and increases the amount of CsrA [24] , which is known to be a negative regulator of biofilm formation in several bacterial species [25] , [26] . It was also reported that cAMP, the reaction product of adenylate cyclase which is regulated by EIIA Glc , and its receptor protein (CRP) directly and indirectly represses the expression of the diguanylate cyclase CdgA, which positively regulates biofilm formation in the V. cholerae C1552 strain [20] , [27] . While the exogenous addition of cAMP represses the biofilm formation also in the V. cholerae MO10 strain, EIIA Glc was shown to activate biofilm formation in the presence of exogenous cAMP in this strain [28] . Collectively, these findings suggest the additional regulatory role of EIIA Glc on biofilm formation. Here, we explored the molecular mechanism of how the biofilm formation is affected by carbon sources in V. cholerae . We find that EIIA Glc interacts with and modulates the activity of a c-di-GMP phosphodiesterase (PDE) depending on its phosphorylation state and thereby regulates biofilm formation in the aquatic and host environment. We propose that EIIA Glc functions as a PTS sugar-responsive regulator of the c-di-GMP-signaling pathway and determines whether to disperse from or stay in the biofilm in response to carbohydrates. EIIA Glc interacts with an EAL domain-containing protein in V. cholerae In many bacteria, EIIA Glc has been implicated in various sugar-dependent regulatory functions [13] . While it was suggested that EIIA Glc participates in the regulation of biofilm formation in the presence of PTS carbohydrates in V. cholerae [9] , [15] , no operative mechanisms were yet offered. To examine the effects of EIIA Glc on biofilm formation, we measured biofilm production in the presence and absence of glucose. While wild-type V. cholerae had a higher level of biofilm formation in the presence of glucose than its absence, which was consistent with previous reports [29] , [30] , a crr -deficient mutant exhibited no difference between the two conditions (Fig. 1a ). Interestingly, while the crr mutant had a similar growth (Supplementary Fig. 1 ), this mutant exhibited a higher level of biofilm formation compared to the wild-type strain in LB medium (Fig. 1a ), which is contrary to a previous study [9] . The exogenous addition of cAMP did not significantly alter the sugar effect, indicating that the regulation of biofilm formation by EIIA Glc is independent of cAMP. These results led us to search for the regulator of biofilm formation, which transduces the sugar signal by directly interacting with EIIA Glc in V. cholerae . Fig. 1 Specific interaction of VC1710 with EIIA Glc . a The biofilm-forming activity of wild-type V. cholerae N16961 and an otherwise isogenic Δ crr mutant was measured in LB alone or supplemented with glucose or glucose and cAMP, as indicated. Biofilm formation was assessed following the static growth of V. cholerae cells for 23 h using a crystal violet staining method [61] , [62] . The stained biofilm formation was determined at 550 nm. Statistical significance was assessed using Student’s t -test ( p -values > 0.05 were presented, ** p -value < 0.01). Shown are the means and SD ( n = 3, independent measurements). b Ligand fishing experiment was carried out to find proteins interacting with His-EIIA Glc . Crude extract prepared from V. cholerae O1 biovar El Tor N16961 cells was mixed with buffer A (lane 1) or 100 μg of purified His-EIIA Glc (lanes 2 and 3). The extract containing His-EIIA Glc was supplemented with either 2 mM glucose to dephosphorylate EIIA Glc (lane 2) or 2 mM PEP to phosphorylate EIIA Glc (lane 3). Each mixture was subjected to TALON metal affinity chromatography and proteins bound to the column were analyzed as described in the “Methods” section. c A mixture of E. coli cell lysates expressing recombinant VC1710 and VCA1085 ( V. cholerae FapA) (lane CE) was mixed with buffer A or His-EIIA Glc and subjected to TALON metal affinity chromatography as in panel b . d The binding affinities of VC1710 with either dephosphorylated (black square) or phosphorylated EIIA Glc (white square) were measured using NanoTemper Monolith NT.115 pico . The dissociation constants ( K d ) of VC1710 complexed with dephosphorylated and phosphorylated EIIA Glc (P~EIIA Glc ) were obtained from three technical replicates. Shown are the means and SD ( n = 3, independent measurements). Full size image To find a new interaction partner of EIIA Glc , we performed ligand fishing experiments using hexahistidine-tagged EIIA Glc (His-EIIA Glc ) as bait [22] . Total proteins extracted from wild-type V. cholerae O1 biovar El Tor N16961 cells grown overnight at 37 °C were mixed with TALON metal-affinity resin in the absence and presence of purified His-EIIA Glc . His-EIIA Glc was dephosphorylated by adding glucose or phosphorylated by adding PEP to the mixtures. After several washes, total proteins bound to the resins were eluted with 200 mM imidazole and analyzed by SDS–PAGE and staining with Coomassie brilliant blue R (Fig. 1b ). In repeated experiments, we could find three protein bands migrating with apparent molecular masses of approximately 100, 90, and 60 kDa, respectively, that were significantly and reproducibly enriched in the fraction containing both His-EIIA Glc and glucose (lane 2). Peptide mapping of these proteins following in-gel tryptic digestion revealed that the protein band migrating at ~100 kDa corresponded to VC2072, an ortholog of the insulin-degrading enzyme IDE (VcIDE) [31] , and the band at ~60 kDa to VCA1085, an ortholog of the flagella assembly protein FapA (VcFapA) [22] . Since IDE and FapA were already reported to interact with EIIA Glc in V. vulnificus [22] , [31] , the elution of the two proteins only in the fraction containing His-EIIA Glc indicates the reliability of this ligand fishing method (compare lanes 1 and 2). Interestingly, the band at ~90 kDa was identified as a putative EAL domain-containing c-di-GMP PDE encoded by vc1710 . The EAL domain is responsible for degrading bis-(3′–5′)-cyclic diguanosine monophosphate (c-di-GMP) to pGpG [32] , which is known to repress biofilm formation and induce biofilm dispersion. Thus, we assumed that the interaction of EIIA Glc with this EAL domain protein might be implicated in biofilm formation as a response to the sugar signal. Interactions of a PTS component with its target proteins are usually dependent on the phosphorylation state of that PTS component. While the specific interaction between IDE and EIIA Glc was reported to be independent of the phosphorylation state of EIIA Glc [31] , FapA was shown to interact only with dephosphorylated EIIA Glc in V. vulnificus [22] . In accordance with these previous studies, VcFapA was not co-eluted with His-EIIA Glc in the fraction incubated with PEP (lane 3 in Fig. 1b ), while the VcIDE band was clearly detected in the eluted fraction containing phosphorylated His-EIIA Glc . Since VC1710 band was detected in the two fractions incubated with EIIA Glc and either glucose or PEP, we assumed that VC1710 interacts with both dephosphorylated and phosphorylated EIIA Glc . To validate the ligand-fishing data, His-EIIA Glc , EI, and HPr was mixed with glucose or PEP, and the phosphorylation state of His-EIIA Glc was confirmed by its mobility shift in an SDS–PAGE gel first [33] . Then a mixture of E. coli cell extracts expressing recombinant VC1710 and VcFapA (lane CE) was added and subjected to protein affinity pull-down assays to determine their interaction with either form of EIIA Glc (lanes 2 and 3 in Fig. 1c ). As expected, while VcFapA interacted only with dephosphorylated EIIA Glc , VC1710 appeared to interact with both the dephosphorylated and phosphorylated forms of EIIA Glc . For quantitative analysis of the binding affinity of VC1710 for EIIA Glc , the dissociation constants ( K d ) of VC1710 complexed with dephosphorylated and phosphorylated EIIA Glc (P~EIIA Glc ) were measured by microscale thermophoresis (MST) experiments. VC1710 showed a slightly higher affinity toward the dephosphorylated form of EIIA Glc ( K d = 114.1 ± 13.7 nM) than toward phosphorylated EIIA Glc (286.7 ± 39.5 nM) (Fig. 1d ). This tight interaction of VC1710 with EIIA Glc led us to assume that the physiological form of VC1710 exists as a complex with EIIA Glc and the activity of VC1710 can be influenced by the phosphorylation state of EIIA Glc , as exemplified by the interaction of adenylate cyclase with EIIA Glc in E. coli [17] . EIIA Glc regulates c-di-GMP PDE activity of VC1710 An analysis of the primary structure of VC1710 indicated that this protein consists of a PAS-sensing domain in the N-terminus and an EAL domain predicted to encode a c-di-GMP PDE in the C-terminus [34] . It has also been previously reported that VC1710 binds c-di-GMP [35] , suggesting its function in c-di-GMP metabolism. To determine whether VC1710 possesses PDE activity, we purified VC1710 and performed an in vitro PDE activity assay by reverse-phase HPLC. The concentration of remaining c-di-GMP decreased with a concomitant increase in the product pGpG after incubation with VC1710, and we could therefore confirm that VC1710 exhibited the predicted c-di-GMP hydrolytic activity (Fig. 2a, b ). Then, to investigate if the PDE activity of VC1710 was affected by its interaction with EIIA Glc , dephosphorylated or phosphorylated EIIA Glc was added to the reaction mixture. The phosphorylation states of EIIA Glc could be successfully modulated by incubation with EI, HPr, and PEP, as shown in the SDS–PAGE analysis (Fig. 2c ). When phosphorylated EIIA Glc was mixed with VC1710, the PDE activity was higher than that in the absence of EIIA Glc . However, no c-di-GMP was digested in the reaction incubated with dephosphorylated EIIA Glc , suggesting that dephosphorylated EIIA Glc inactivates the PDE activity of VC1710. To elucidate the kinetic properties of the VC1710 protein, we determined K m and V max values based on three independent activity assays. When c-di-GMP was reacted with VC1710 alone, the K m value was ~4.58 μM. However, when phosphorylated EIIA Glc was added to the VC1710 reaction mixture, the K m value for c-di-GMP decreased to 1.30 μM (Supplementary Fig. 2 ). Given that the K d values for c-di-GMP - binding proteins ranged up to several μM and the K m values of PDEs ranged from 60 nM to several μM [36] , the K m values of VC1710 for c-di-GMP appear to be biochemically and physiologically relevant to the control of the c-di-GMP level and thereby related phenotypes in vivo. To exclude the possibility of carrier protein effect, we performed the same experiment without EIIA Glc or in the presence of the same amount of BSA, and no measurable effect was detected (Supplementary Fig. 3 ). The analytical western blot data (Supplementary Fig. 4 ) shows that the number of the EIIA Glc protein in a V. cholerae cell is more than 100 times higher than that of the VC1710 protein. We, therefore, conclude that VC1710 is always present in a complex form with EIIA Glc in the cell and that the activity of VC1710 is entirely dependent on the phosphorylation state of EIIA Glc . As the phosphorylation state of EIIA Glc was altered in response to the type of sugars [11] , we named VC1710 as PdeS (for S ugar-responsive PDE). Fig. 2 EIIA Glc modulates the PDE activity of VC1710. a The c-di-GMP phosphodiesterase (PDE) activity of VC1710 (4.1 μM) was assayed in a reaction mixture containing 20 μM of c-di-GMP and 0.4 μM of EI and HPr in the absence or presence of purified EIIA Glc (17.1 μM). EIIA Glc in the reaction mixture was phosphorylated by adding 2 mM PEP. The reaction mixtures were applied to a Supercosil LC-18-T HPLC column, and the remaining c-di-GMP and produced pGpG were quantified by measuring absorbance at 254 nm. b The c-di-GMP hydrolysis activity of VC1710 was assessed in the absence (black square) and presence of EIIA Glc (white and gray squares) as in panel a and c-di-GMP and pGpG were analyzed at 0, 10, 30, 60, 180, and 300 s. c The phosphorylation state of EIIA Glc in panels a and b was confirmed by SDS–PAGE and staining with Coomassie brilliant blue R. d The binding affinities of PdeS with c-di-GMP in the absence (black square) or presence (white square) of dephosphorylated EIIA Glc were measured using NanoTemper Monolith NT.115 pico . An excess amount (5 μM) of EIIA Glc was added to the reaction mixture to ensure all the VC1710 existed as a complex with EIIA Glc . Shown are the means and SD ( n = 3, independent measurements). Full size image From the MST assay, we could measure the dissociation constant of the PdeS/c-di-GMP complex to be ~8.7 μM (Fig. 2d ), which is comparable with the K m value of PdeS toward c-di-GMP. Interestingly, however, we could not detect any interaction of c-di-GMP with PdeS in the presence of dephosphorylated EIIA Glc , indicating that PdeS becomes inaccessible to c-di-GMP when it forms a complex with the dephosphorylated form of EIIA Glc (Fig. 2d ). Therefore, it could be assumed that the tight binding of dephosphorylated EIIA Glc inactivates the PDE activity of PdeS by blocking the accessibility of c-di-GMP to the active site. EIIA Glc regulates the activity of PdeS in vivo To test whether PdeS can also digest c-di-GMP in the cell, we compared intracellular concentrations of c-di-GMP between the wild-type and a pdeS -deficient mutant strain (Δ pdeS ) of V. cholerae N16961 (Fig. 3a ). Because EIIA Glc in cells growing in LB medium is mostly in its phosphorylated form (Fig. 4a ), which stimulates the PDE activity of PdeS, the cells grown in the buffered LB medium were used to extract c-di-GMP. Measurement using LC–MS/MS revealed that Δ pdeS cells had an ~2.5-fold higher concentration of c-di-GMP than wild-type cells as expected. In addition, the Δ pdeS strain had a higher expression level of the Vibrio polysaccharide synthesis ( vps ) operon and thus formed significantly more biofilm than the wild-type strain, which is consistent with previous reports showing that c-di-GMP induces biofilm formation [37] , [38] (Fig. 3a, b ; Supplementary Fig. 5a ). We found that an alanine substitution mutant in the EAL domain of PdeS (PdeS(E450A)) resulted in the complete abolishment of the PDE activity (Supplementary Fig. 3 ). While the Δ pdeS strain carrying an expression vector for wild-type PdeS exhibited similar levels of biofilm formation and vps expression with those of the wild-type strain, the mutant strain expressing PdeS(E450A) did not complement these phenotypic changes (Supplementary Figs. 5b and 6 ). Thus, we concluded that PdeS regulates biofilm formation through its PDE activity. Fig. 3 PdeS regulates the c-di-GMP level and biofilm formation. a The intracellular c-di-GMP concentration and the biofilm-forming activity of wild-type N16961 and a Δ pdeS strain were measured in the buffered LB medium. The concentration of c-di-GMP extracted from the V. cholerae cells was determined using LC–MS/MS, and normalized with total protein contents. Biofilm formation was assessed following static growth of V. cholerae cells for 23 h using a crystal violet staining method [61] , [65] . The biofilm formation was determined at 550 nm. b Biofilm formation was visualized using confocal laser scanning microscopy. Scale bar: 50 μm. c The effect of EIIA Glc on the c-di-GMP hydrolysis activity of PdeS was assessed in vivo. The intracellular c-di-GMP concentration and the biofilm-forming activity of wild-type and Δ pdeS V. cholerae strains harboring a pBAD-based expression vector for either wild-type EIIA Glc or dephosphomimetic mutant EIIA Glc (H91A) were determined in the presence of 0.1% arabinose as described in panel a . Statistical significance was assessed using Student’s t -test ( p- values > 0.05 were presented, * p- value < 0.05, ** p -value < 0.01). Shown are the means and SD ( n = 3, independent measurements). Full size image Fig. 4 PdeS regulates biofilm formation depending on carbon sources. a The level of biofilm formation was compared between wild-type N16961 and a Δ pdeS strain in the presence of various carbon sources in buffered LB medium as in Fig. 3 . At the same time, the phosphorylation state of EIIA Glc was determined by western blot using anti-EIIA Glc mouse serum after SDS–PAGE. Statistical significance was assessed using Student’s t -test (* p- value < 0.05, p- values > 0.05 were presented). Glc, glucose; NAG, N-acetylglucosamine; Mtl, mannitol; Succ, Succinate. b The inhibitory effect of PdeS on the biofilm formation was plotted as a function of EIIA Glc phosphorylation. Based on the data in panel a , the degree of biofilm formation of wild-type cells was divided by that of the Δ pdeS mutant cells. The percentage of biofilm formation inhibition by PdeS was then calculated by subtracting the resultant value from 1 and multiplying by 100, then plotted as a function of the percentage of phosphorylated EIIA Glc over total EIIA Glc . The correlation between the sugar-mediated phosphorylation state of EIIA Glc and biofilm formation was assessed using Pearson’s correlation coefficient ( r = 0.9242, p < 0.005). Shown are the means and SD ( n = 3, independent measurements). Full size image Then, to confirm whether the regulation of the PdeS activity by EIIA Glc also operates in V. cholerae cells, we constructed a dephosphomimetic mutant (H91A) of crr encoding EIIA Glc on the chromosome and performed biofilm formation assays (Supplementary Fig. 7a ). While we observed that the dephosphomimetic crr mutant showed increased biofilm formation compared to the wild-type strain, this stimulatory effect was not observed in a pdeS deletion mutant. EIIA Glc is shared for several membrane-bound enzyme IIBCs including those specific for glucose, N -acetylglucosamine, sucrose, and trehalose in V. cholerae [9] and phosphorylatable EIIA Glc is indispensable for a variety of physiological processes including the regulation of global transcription factors such as CRP and Mlc. Therefore, we assume that the phenotype of this chromosomal crr mutant might be due to indirect pleiotropic effects of the mutation. For this reason, we tried to see the effect of EIIA Glc dephosphorylation on biofilm formation by increasing the level of the dephosphomimetic mutant of EIIA Glc , while minimizing the perturbation of the overall PTS activity. Therefore, we compared biofilm formation and the intracellular level of c-di-GMP of the wild-type strain carrying an expression vector for wild-type EIIA Glc with the wild-type strain carrying an expression vector for EIIA Glc (H91A), and observed increased biofilm formation and the c-di-GMP level in the latter strain (Fig. 3c ; Supplementary Fig. 7 ), which is in accordance with the result obtained by the chromosomal mutation of the crr gene. Together our data show that dephosphorylated EIIA Glc inactivates the PDE activity of PdeS and thereby increases the c-di-GMP level in vivo. Thus, it could be assumed that EIIA Glc can modulate biofilm formation by controlling the c-di-GMP level through direct interaction with PdeS. EIIA Glc regulates biofilm formation depending on carbon sources PTS components including EIIA Glc can have a different phosphorylation state depending on the availability of PTS substrates. As the PDE activity of PdeS and thus the intracellular concentration of c-di-GMP are modulated depending on the phosphorylation state of EIIA Glc , we examined whether biofilm formation can be influenced by carbohydrates encountered by V. cholerae in their environmental niches. Thus, we performed a biofilm formation assay in the presence of various carbon sources in LB medium. To exclude the effect of the pH decrease due to fermentation of sugar, we buffered LB medium with 40 mM potassium phosphate, pH 7.0. At the same time, we determined the in vivo phosphorylation state of EIIA Glc in each medium (Fig. 4a ). Consistent with previously reported results in E. coli and V. vulnificus [11] , [22] , EIIA Glc was mostly dephosphorylated in glucose-containing medium, while mostly phosphorylated in LB medium without additional carbon source. We could also find a significant positive correlation between the degree of EIIA Glc phosphorylation and the inhibitory effect of PdeS on biofilm formation (Fig. 4b ). These data imply that the modulation of biofilm formation by PdeS is dependent on the phosphorylation state of EIIA Glc , which is determined by the environmental carbon source. EIIA Glc regulates biofilm formation and host gut colonization V. cholerae is associated with various hosts, including arthropods, insect eggs, and unicellular eukaryotes as well as humans [39] . Recently, the interaction between V. cholerae and the fruit fly Drosophila melanogaster has been intensively studied, since this arthropod model acts as a disease reservoir in nature [40] and is also simple but has similar physiological features and anatomical structures with mammalian infection models [41] . It has been reported that Vibrio exopolysaccharide (VPS)-dependent biofilm formation is indispensable for attachment and colonization in the Drosophila intestine in a quorum sensing-defective V. cholerae strain [42] , [43] . Therefore, we assumed that VPS might also play a critical role in the intestinal colonization in the N16961 strain which carries a natural frame-shift mutation in the hapR gene encoding the quorum-sensing master regulator HapR. As the expression of the vps operon was controlled by c-di-GMP, which is the substrate of PdeS, we assumed that PdeS might also play a role in the regulation of intestinal colonization. Since mannitol transport by V. cholerae requires mannitol-specific EII but not EIIA Glc in spite of its structural similarity with glucose, the phosphorylation state of EIIA Glc is different in the presence of the two PTS sugars (Fig. 4a ). Therefore, we chose glucose and mannitol as representative sugars leading to dephosphorylation and ~50% phosphorylation of EIIA Glc , respectively, to evaluate the EIIA Glc phosphorylation state-dependent regulation of the colonization efficiency of V. cholerae . To investigate whether a sugar-dependent change in EIIA Glc phosphorylation influences bacterial colonization in the intestine through the modulation of PdeS activity, flies were fed 5% sugar (glucose or mannitol) solution containing ~10 6 cells μl −1 of the V. cholerae N16961 strain for 24 h, and subsequently fed the same sugar solution without bacteria for 9 h. These flies were then surface-sterilized, homogenized in 1 ml of PBS buffer and spread on an agar plate for the quantification of the colonization of V. cholerae in vivo by measuring colony-forming units (CFUs). While the CFU of the Δ pdeS strain was not affected by the sugar source, the CFU of the wild-type strain was significantly lower in flies fed mannitol compared to flies fed glucose (Fig. 5a ). In flies fed mannitol, the wild-type strain gave significantly lower CFU levels compared to the Δ pdeS strain. Therefore, we could assume that, in the presence of mannitol, phosphorylated EIIA Glc stimulates the PdeS activity to decrease the c-di-GMP level and thereby biofilm formation. Fig. 5 PdeS regulates intestinal colonization depending on the host diet. a Flies were orally administered a 5% sugar solution containing the indicated V. cholerae strains for 24 h, and fed a sterile sugar solution for another 9 h. The homogenate of the surface-sterilized fly was spread on a selective medium for V. cholerae and colony-forming units (CFU) were measured. b Intestinal colonization was assessed for a shorter infection period. Flies were orally administered a 5% sugar solution containing the indicated V. cholerae strains for 2 h, and fed a sterile sugar solution for another 2 h. c The V. cholerae colonization on the alimentary canal was visualized using confocal laser scanning microscopy. Flies were exposed to V. cholerae strains harboring a GFP expression vector in the presence of 5% mannitol for 2 h and, after incubation in a sterile medium for another 2 h, the whole intestines were dissected and visualized. Shown are the representative images from three independent experiments on different days. Scale bar: 500 μm. d Food consumption was measured by dye uptake using FD&C Blue #1 dye during bacterial infection [64] . Shown are the means and SD ( n = 6, independent measurements). Data was analyzed using a two-way ANOVA followed by Tukey’s post hoc test (* p -value < 0.05, *** p -value < 0.005, p- values > 0.05 were presented). Full size image To determine whether the effect of PdeS on intestinal colonization is mediated by the regulation of biofilm formation, we repeated the colonization experiment with Δ vpsA and Δ vpsA pdeS mutants (Fig. 5a ). As reported previously [42] , [43] , mutation of vpsA resulted in a significantly reduced (~5%) intestinal colonization in flies compared to the wild-type strain. Interestingly, the inhibitory effect of PdeS on intestinal colonization was not seen in this vpsA -mutant strain. Thus, it could be assumed that VPS-dependent biofilm formation is important for the regulation of intestinal colonization by PdeS. Then, to assess whether PdeS affects the earlier stage of V. cholerae infection of the Drosophila intestine, we infected flies orally with 5% sugar solution containing ~10 8 cells μl −1 of wild-type V. cholerae N16961 or its pdeS mutant for 2 h. After feeding flies with bacteria-free 5% sugar solution for another 2 h and surface sterilization, we quantified the intestinal colonization of V. cholerae by measuring CFUs (Fig. 5b ). While the CFU of the Δ pdeS strain showed no difference depending on the sugar source, the CFU of the wild-type strain was significantly lower in flies fed mannitol compared to flies fed glucose. Therefore, our data indicates that PdeS may regulate the initial phase of intestinal colonization of V. cholerae . To determine which compartment(s) V. cholerae colonizes and to examine the physiological relevance of the host diet-dependent colonization, flies were exposed to the V. cholerae N16961 strain carrying a GFP expression vector in the presence of 5% mannitol, and their colonization on the whole alimentary canal was visualized (Fig. 5c ). Although the amounts of ingested bacteria (as estimated by the ingested amounts of bacteria-containing sugar solutions) were similar between wild-type and Δ pdeS strains (Fig. 5d ), more intensive colonization was detected in flies infected with the Δ pdeS strain than in flies infected with the wild-type strain, especially in the anterior midgut, which is the main site of digestion and nutrient absorption [44] in our infection condition (Fig. 5c ). This result is consistent with the CFU data (Fig. 5b ), implying that PdeS modulates the colonization efficiency of V. cholerae depending on the host diet, which is consistent with its sugar-dependent regulation of c-di-GMP and biofilm formation. The pathogen Vibrio cholerae , like other bacteria, has various niches including natural seawater, copepod, chironomid egg masses, and the human host [39] . The ability to sense and respond to each environment is the crucial factor for adaptation and propagation of bacteria. In many bacteria, the PTS is one of the sensory systems that regulate multiple metabolic pathways in response to the availability of carbon or nitrogen nutrients in diverse environments [45] . Previous studies suggested that the PTS in V. cholerae also has regulatory functions in biological processes, such as biofilm formation [14] , [28] , colonization in the mammal host [9] , chitin utilization, and natural competence [46] . Because most of these regulations are mediated by protein–protein interactions [13] , the characterization of the interaction network of the PTS is vital for understanding the orchestrated cellular responses to environmental changes. In this study, we found a new interaction partner of EIIA Glc , the c-di-GMP PDE PdeS which hydrolyzes the ubiquitous bacterial second messenger c-di-GMP. As the c-di-GMP-signaling pathway is involved in many behaviors, such as biofilm formation, motility, and toxin production, this interaction is expected to be an important key to reveal many nutrient-related phenotypes. Many studies suggested that c-di-GMP induces the transition from motile to sessile mode by binding to and regulating various receptors involved in biofilm formation [27] , [47] . Biofilm matrix serves as a barrier against various environmental stresses, which enables bacteria to prosper as long as sufficient nutrients are available. However, once nutrients become scarce, bacterial cells detach and disperse from this community by reducing the production of this polymeric matrix. Several studies have reported that nutrient deprivation decreases biofilm formation and induces biofilm dispersion by decreasing intracellular c-di-GMP [48] , [49] , [50] . The interaction between EIIA Glc and PdeS is expected to be one of these regulatory mechanisms. It is notable that modulation of c-di-GMP hydrolytic activity of PdeS by EIIA Glc is comparable to the regulation of cAMP synthetic activity of adenylate cyclase [17] . In several bacteria, only the phosphorylated form of EIIA Glc is known to stimulate cAMP synthesis [13] , [17] , [22] . Similarly, our data in this study show that dephosphorylated EIIA Glc strongly inhibits c-di-GMP hydrolysis, whereas its phosphorylated form stimulates c-di-GMP hydrolysis in V. cholerae . The copy number of the EIIA Glc protein was reported to be 20,000–30,000, while that of adenylate cyclase to be <10 in E. coli [51] . According to our analytical western blot results, the copy number of EIIA Glc in a V. cholerae cell was estimated to be similar to that in E. coli and that of the PdeS protein to be 29–153 (Supplementary Fig. 4 ). Because the number of EIIA Glc is significantly higher than that of PdeS and adenylate cyclase, EIIA Glc appears to simultaneously control the amount of c-di-GMP and cAMP, yet in the opposite direction, in V. cholerae . As the cAMP-CRP complex has been reported to inhibit biofilm formation by differentially regulating the expression of several c-di-GMP-metabolizing enzymes [18] , [20] , it was expected that the cAMP pathway would mitigate the regulatory effect of PdeS on biofilm formation. However, the expression level of PdeS was not changed by the sugar type (Supplementary Fig. 8 ). Moreover, the PdeS-mediated regulation of biofilm formation was quantitatively correlated to the phosphorylation state of EIIA Glc (Fig. 4 ). Therefore, we concluded that although the intracellular level of cAMP and c-di-GMP was controlled at the same time, the sugar-dependent c-di-GMP-regulatory pathway is hardly affected by the cAMP-signaling pathway in V. cholerae N16961. In addition, it could be assumed that the indirect interplay between the cAMP and c-di-GMP-signaling pathways might play only a minor role, if any, in the sugar-dependent regulation of biofilm formation in this strain. In previous studies, different effects of cAMP–CRP on biofilm formation have been reported among various V. cholerae strains. While biofilm formation was negatively regulated by the cAMP–CRP complex in the C1552 and C6728 strains [20] , [52] , the supplementation of the growth medium with various concentrations of cAMP had no effect on the total growth and biofilm accumulation by a crr mutant of the MO10 strain [28] . Herein, we report that the sugar-dependent regulation of biofilm formation is not affected by cAMP–CRP in the N16961 strain. This may simply be the result of strain differences, as V. cholerae is known to undergo genetic drift in laboratory culture [53] . During the host infection, the intracellular concentration of c-di-GMP in V. cholerae is changed along its infection stage [54] . Also, the c-di-GMP pool fluctuates in response to various external signals, choosing the fittest infection strategy depending on the environmental condition [55] . Thus, the sophisticated regulation of c-di-GMP contents appears to be a prerequisite for a successful propagation and transmission to new hosts throughout the infection cycle. In this respect, our findings provide a new insight into how pathogenic bacteria cope with fluctuating nutritional conditions including those encountered during passage through the intestinal tract of the host. 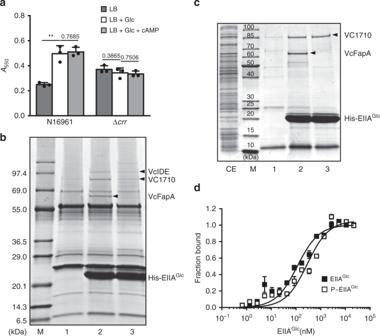Fig. 1 Specific interaction of VC1710 with EIIAGlc.aThe biofilm-forming activity of wild-typeV. choleraeN16961 and an otherwise isogenic Δcrrmutant was measured in LB alone or supplemented with glucose or glucose and cAMP, as indicated. Biofilm formation was assessed following the static growth ofV. choleraecells for 23 h using a crystal violet staining method61,62. The stained biofilm formation was determined at 550 nm. Statistical significance was assessed using Student’st-test (p-values > 0.05 were presented, **p-value < 0.01). Shown are the means and SD (n= 3, independent measurements).bLigand fishing experiment was carried out to find proteins interacting with His-EIIAGlc. Crude extract prepared fromV. choleraeO1 biovar El Tor N16961 cells was mixed with buffer A (lane 1) or 100 μg of purified His-EIIAGlc(lanes 2 and 3). The extract containing His-EIIAGlcwas supplemented with either 2 mM glucose to dephosphorylate EIIAGlc(lane 2) or 2 mM PEP to phosphorylate EIIAGlc(lane 3). Each mixture was subjected to TALON metal affinity chromatography and proteins bound to the column were analyzed as described in the “Methods” section.cA mixture ofE. colicell lysates expressing recombinant VC1710 and VCA1085 (V. choleraeFapA) (lane CE) was mixed with buffer A or His-EIIAGlcand subjected to TALON metal affinity chromatography as in panelb.dThe binding affinities of VC1710 with either dephosphorylated (black square) or phosphorylated EIIAGlc(white square) were measured using NanoTemper Monolith NT.115pico. The dissociation constants (Kd) of VC1710 complexed with dephosphorylated and phosphorylated EIIAGlc(P~EIIAGlc) were obtained from three technical replicates. Shown are the means and SD (n= 3, independent measurements). Bacterial strains, plasmids, and culture conditions The bacterial strains and plasmids used in this study are listed in Supplementary Table 1 . Construction of the deletion strains was performed as described previously [56] . V. cholerae strains were cultured in Luria-Bertani medium. Purification of overexpressed proteins While EI, HPr, and EIIA Glc were expressed in a ptsHIcrr -deleted E. coli ER2566 strain, other proteins were expressed in wild-type ER2566 by adding 1 mM IPTG. His-tagged proteins were purified using TALON metal-affinity resin (Takara Bio.) according to the manufacturer’s instructions. After His-tagged proteins were eluted with 200 mM imidazole, the fractions containing His-tagged proteins were pooled and concentrated using Amicon Ultracel-3K centrifugal filters (Merck Millipore). To increase the purity of proteins and remove imidazole, the concentrated pool was chromatographed on a Hiload 16/60 Superdex 200 pg column (GE Healthcare) equilibrated with buffer A (25 mM HEPES–NaOH (pH 7.6), containing 100 mM NaCl, 10 mM β-mercaptoethanol, and 10% glycerol). Ligand fishing using metal-affinity beads Ligand-fishing experiments were performed as described previously with minor modifications to find a new interaction partner of EIIA Glc [23] , [57] . V. cholerae O1 biovar El Tor N16961 cells grown at 37 °C overnight at LB (200 ml) were harvested and resuspended in buffer A. Cells were then disrupted by three passages through a French pressure cell at 8000 psi. After centrifugation at 10,000× g for 20 min at 4 °C, the supernatant was mixed with 100 μg of His-EIIA Glc or buffer A as control in the presence of TALON metal-affinity resin in a 15-ml tube, then incubated at 4 °C for 30 min. His-EIIA Glc was dephosphorylated by adding glucose or phosphorylated by adding PEP to the mixtures. After brief washes with buffer A containing 10 mM imidazole, the bound proteins were eluted with buffer A containing 200 mM imidazole and analyzed by SDS–PAGE using a 4–20% gradient Tris–glycine gel (KOMA biotech) and staining with Coomassie brilliant blue R. Protein bands specifically bound to the His-tagged bait protein were excised from the gel, and in-gel digestion and peptide mapping of the tryptic digests were performed using MALDI-TOF MS [57] , [58] . c-di-GMP PDE activity assay using HPLC c-di-GMP PDE activity was determined by measuring the remaining c-di-GMP and produced pGpG after the reaction [59] . The reaction contained 20 mM Tris–HCl (pH 8.0), 50 mM NaCl, 5 mM MgCl 2 , 0.5 mM EDTA, and 20 μM c-di-GMP in addition to PdeS in a total volume of 40 μl. To test the effect of the phosphorylation state of EIIA Glc on PDE activity, EIIA Glc and 0.4 μM of EI and HPr were added in the presence or absence of PEP. The phosphorylation states of EIIA Glc were confirmed by SDS–PAGE and staining with Coomassie brilliant blue R [12] . The enzymatic reaction was started by the addition of c-di-GMP and allowed to proceed at 37 °C. Aliquots of each reaction were taken at appropriate times and reactions were stopped by adding 10 mM CaCl 2 . These mixtures were boiled for 5 min and centrifuged. Then 20 μl of each supernatant was injected into a Supelcosil LC-18-T column (Sigma-Aldrich) using an Agilent HP1200 HPLC system (Agilent Technology). The separations of pGpG and c-di-GMP were performed by gradient elution at a flow rate of 1.0 ml min −1 and chromatograms were recorded at 254 nm. The gradient program was: 0–5 min, isocratic elution with 100 mM potassium phosphate, pH 6.0 (A); 5–13 min, linear gradient to 70% A and 30% methanol (B); 13–16 min, isocratic at B; 16–18 min, linear gradient to A; 18–20 min, isocratic at A. 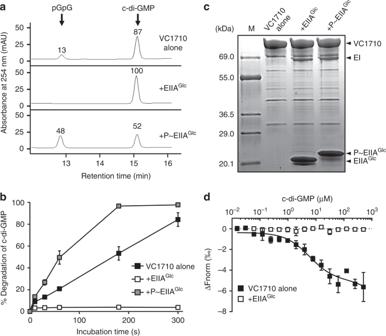Fig. 2 EIIAGlcmodulates the PDE activity of VC1710.aThe c-di-GMP phosphodiesterase (PDE) activity of VC1710 (4.1 μM) was assayed in a reaction mixture containing 20 μM of c-di-GMP and 0.4 μM of EI and HPr in the absence or presence of purified EIIAGlc(17.1 μM). EIIAGlcin the reaction mixture was phosphorylated by adding 2 mM PEP. The reaction mixtures were applied to a Supercosil LC-18-T HPLC column, and the remaining c-di-GMP and produced pGpG were quantified by measuring absorbance at 254 nm.bThe c-di-GMP hydrolysis activity of VC1710 was assessed in the absence (black square) and presence of EIIAGlc(white and gray squares) as in panelaand c-di-GMP and pGpG were analyzed at 0, 10, 30, 60, 180, and 300 s.cThe phosphorylation state of EIIAGlcin panelsaandbwas confirmed by SDS–PAGE and staining with Coomassie brilliant blue R.dThe binding affinities of PdeS with c-di-GMP in the absence (black square) or presence (white square) of dephosphorylated EIIAGlcwere measured using NanoTemper Monolith NT.115pico. An excess amount (5 μM) of EIIAGlcwas added to the reaction mixture to ensure all the VC1710 existed as a complex with EIIAGlc. Shown are the means and SD (n= 3, independent measurements). Determination of the intracellular concentration of c-di-GMP V. cholerae was cultivated in LB medium (100 ml) to OD 600 ~ 1.0, and centrifuged at 4000× g for 10 min. The cell pellet was resuspended in 500 μl extraction buffer (40% methanol, 40% acetonitrile, and 0.1 N formic acid) and incubated on ice for 15 min. Each sample was subjected to three cycles of freezing/thawing using liquid nitrogen and heat block adjusted to 90 °C. After an additional 15-min incubation on ice, the sample was centrifuged at 16,100× g for 10 min, and 400 μl of the supernatant was dried under vacuum. The lyophilized nucleotides were resuspended in 80 μl of distilled water. Quantification of the c-di-GMP was carried out using HPLC coupled with triple quadrupole mass spectrometry. The temperatures of the column oven and autosampler were maintained at 25 and 20 °C, respectively. Ten microliters of the resuspended nucleotides were injected to a Hypersil GOLD HILIC column (2.1 × 100 mm, particle size 1.9 μM, pore size 175 Å, Thermo Scientific) using Accela 1250 UPLC TM system (Thermo Fisher Scientific, USA). Separation of c-di-GMP was performed using the following gradient program: solvent A, 20 mM ammonium acetate adjusted to pH 8.0 with ammonium hydroxide; solvent B, acetonitrile (ACN); flow rate 250 μl min −1 ; gradient condition, 0–2 min (15% B), 2–29 min (15–98% B), 29–33 min (98% B), 33–35 min (98–15% B), 35–45 min (15% B). Xanthosine 3′,5′-cyclic monophosphate (cXMP; BioLog) was used as an internal standard. The retention times for c-di-GMP and cXMP were 21.5 and 16.8 min, respectively. The analyte detection was performed using TSQ Quantum Access Max (Thermo Scientific). Tune parameters for TSQ were as follows: capillary temperature, 300 °C; vaporization temperature, 250 °C; sheath gas pressure, 30 psi; aux gas pressure, 10 psi; positive polarity spray voltage, 4.0 kV. The samples were monitored with SRM scan mode. The SRM settings for c-di-GMP and cXMP were optimized and determined as follows: c-di-GMP: [M + H] + m / z 691 → 152; collision energy, 38 eV; cXMP: [M + H] + m / z 347 → 153, collision energy, 18 eV. The measured intracellular concentration of c-di-GMP was normalized with the protein level. MST analysis The binding affinities of PdeS with EIIA Glc and c-di-GMP were measured using a NanoTemper Monolith NT.115 pico instrument [60] . Purified GST-PdeS was labeled with NT-647 using a Monolith protein-labeling kit and used at a concentration of 4.875 nM. Each unlabeled EIIA Glc and c-di-GMP was titrated in 1:1 serial dilutions in MST-binding buffer (25 mM HEPES–NaOH (pH 7.6), 100 mM NaCl, 5 mM β-mercaptoethanol, 0.5 mg ml −1 BSA, 0.05 (v/v) % Tween 20), with the highest concentration of EIIA Glc at 21.9 μM and c-di-GMP at 500 μM. 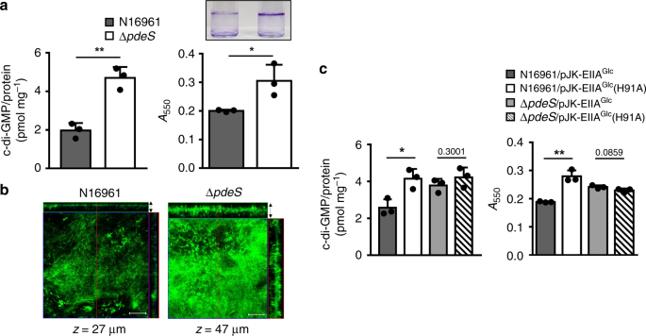Fig. 3 PdeS regulates the c-di-GMP level and biofilm formation.aThe intracellular c-di-GMP concentration and the biofilm-forming activity of wild-type N16961 and a ΔpdeSstrain were measured in the buffered LB medium. The concentration of c-di-GMP extracted from theV. choleraecells was determined using LC–MS/MS, and normalized with total protein contents. Biofilm formation was assessed following static growth ofV. choleraecells for 23 h using a crystal violet staining method61,65. The biofilm formation was determined at 550 nm.bBiofilm formation was visualized using confocal laser scanning microscopy. Scale bar: 50 μm.cThe effect of EIIAGlcon the c-di-GMP hydrolysis activity of PdeS was assessed in vivo. The intracellular c-di-GMP concentration and the biofilm-forming activity of wild-type and ΔpdeS V. choleraestrains harboring a pBAD-based expression vector for either wild-type EIIAGlcor dephosphomimetic mutant EIIAGlc(H91A) were determined in the presence of 0.1% arabinose as described in panela. Statistical significance was assessed using Student’st-test (p-values > 0.05 were presented, *p-value < 0.05, **p-value < 0.01). Shown are the means and SD (n= 3, independent measurements). 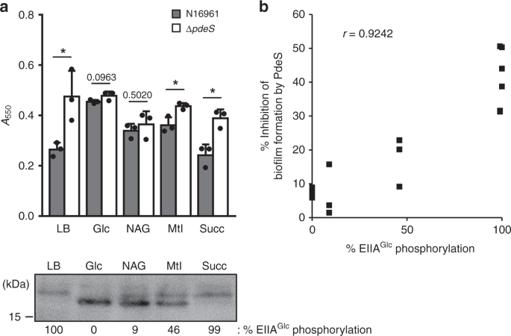Fig. 4 PdeS regulates biofilm formation depending on carbon sources.aThe level of biofilm formation was compared between wild-type N16961 and a ΔpdeSstrain in the presence of various carbon sources in buffered LB medium as in Fig.3. At the same time, the phosphorylation state of EIIAGlcwas determined by western blot using anti-EIIAGlcmouse serum after SDS–PAGE. Statistical significance was assessed using Student’st-test (*p-value < 0.05,p-values > 0.05 were presented). Glc, glucose; NAG, N-acetylglucosamine; Mtl, mannitol; Succ, Succinate.bThe inhibitory effect of PdeS on the biofilm formation was plotted as a function of EIIAGlcphosphorylation. Based on the data in panela, the degree of biofilm formation of wild-type cells was divided by that of the ΔpdeSmutant cells. The percentage of biofilm formation inhibition by PdeS was then calculated by subtracting the resultant value from 1 and multiplying by 100, then plotted as a function of the percentage of phosphorylated EIIAGlcover total EIIAGlc. The correlation between the sugar-mediated phosphorylation state of EIIAGlcand biofilm formation was assessed using Pearson’s correlation coefficient (r= 0.9242,p< 0.005). Shown are the means and SD (n= 3, independent measurements). 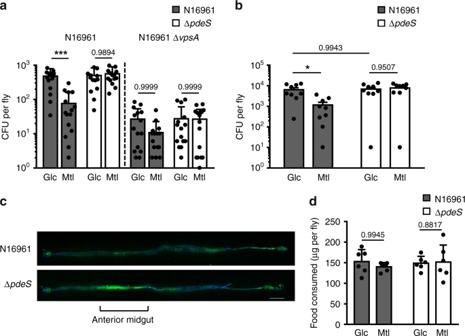Fig. 5 PdeS regulates intestinal colonization depending on the host diet.aFlies were orally administered a 5% sugar solution containing the indicatedV. choleraestrains for 24 h, and fed a sterile sugar solution for another 9 h. The homogenate of the surface-sterilized fly was spread on a selective medium forV. choleraeand colony-forming units (CFU) were measured.bIntestinal colonization was assessed for a shorter infection period. Flies were orally administered a 5% sugar solution containing the indicatedV. choleraestrains for 2 h, and fed a sterile sugar solution for another 2 h.cTheV. choleraecolonization on the alimentary canal was visualized using confocal laser scanning microscopy. Flies were exposed toV. choleraestrains harboring a GFP expression vector in the presence of 5% mannitol for 2 h and, after incubation in a sterile medium for another 2 h, the whole intestines were dissected and visualized. Shown are the representative images from three independent experiments on different days. Scale bar: 500 μm.dFood consumption was measured by dye uptake using FD&C Blue #1 dye during bacterial infection64. Shown are the means and SD (n= 6, independent measurements). Data was analyzed using a two-way ANOVA followed by Tukey’s post hoc test (*p-value < 0.05, ***p-value < 0.005,p-values > 0.05 were presented). To prevent degradation of c-di-GMP by PdeS during the assay, their interaction was examined in the buffer without divalent cations which are indispensable for the PDE activity of PdeS. The measurements were performed at 15% LED power and 30% MST power at 22 °C. Measurement of biofilm formation Overnight-grown cells were inoculated in LB medium buffered with 40 mM potassium phosphate (pH 7.0) in the absence or presence of sugar and incubated under static conditions in a borosilicate tube at 37 °C for 23 h. After planktonic cells were washed away with PBS, the remaining biofilm-associated cells were stained with 0.1% crystal violet (CV) for 20 min. After rinses with PBS three times, the CV-stained biofilm was solubilized with 95% ethanol and measured at 550 nm [61] , [62] . Mature biofilm was also visualized as described previously [63] using confocal laser scanning microscopy (LSM700, Zeiss). V. cholerae strains constitutively expressing green fluorescent protein (GFP) were used for biofilm imaging. Determination of the phosphorylation state of EIIA Glc The phosphorylation state of EIIA Glc was determined as described previously [12] , [33] with some modifications. A 0.2-ml aliquot of cell culture was quenched at OD 600 ~ 0.5 by adding 20 μl of 5 M NaOH followed by vortexing for 15 s, and then 150 μl of 3 M sodium acetate (pH 5.3) and 0.9 ml of ethanol were sequentially added. After incubated at −80 °C for 30 min, each sample was centrifuged at 10,000× g at 4 °C for 30 min, and the pellet was resuspended in 40 μl of SDS sample buffer. A 20-μl aliquot of each sample was then resolved by SDS–PAGE using a 4–20% gradient gel, and EIIA Glc was visualized by western blot using anti-EIIA Glc serum [11] . Measurement of the cellular protein level by western blot A V. cholerae strain in which the chromosomal vc1710 was tagged with 3xFLAG at its C-terminus was grown in LB medium and aliquots were harvested when OD 600 reached 0.4, 1.0, and 1.5, respectively. After the pellets were resuspended in SDS-loading buffer, cells were lysed by boiling for 5 min. Cell lysates were electrophoresed on a SDS–PAGE gel with various amounts of purified VC1710::3xFLAG protein or EIIA Glc as control. For immunodetection, monoclonal mouse anti-FLAG antibody (Sigma-Aldrich) or anti-EIIA Glc mouse serum was used. Uncropped blot images were provided as a source data file. Quantification of V. cholerae colonization in the fly intestine To establish whether sugars could affect the gut colonization of V. cholerae strains, fasted adult flies ( Drosophila melanogaster w1118) were orally administered a 5% sugar solution containing ~10 6 cells μl −1 of the V. cholerae strains in the presence of either glucose or mannitol for 24 h, and fed the same, but sterile, medium for another 9 h. After each fly was immersed in 70% ethanol for 3 min, the surface-sterilized fly was homogenized in 1 ml of sterile PBS and spread on LB agar plates containing 10 μg ml −1 of streptomycin to determine CFUs of V. cholerae . To image bacterial infection, the whole alimentary canal was dissected at the same time point, and visualized by confocal laser scanning microscopy. For measurement of food consumption, the feeding assay was performed with a standard method using FD&C Blue #1 dye [64] . Flies were orally administered a 5% sugar (glucose or mannitol) solution containing V. cholerae cells and 0.5% (w/v) FD&C #1 dye for 2 h. Guts dissected from five flies were homogenized in 200 μl of PBS and the homogenate were centrifuged at 8000× g for 10 min. Food consumption was quantified by measuring absorbance of the supernatant at 625 nm. Reporting summary Further information on research design is available in the Nature Research Reporting Summary linked to this article.